Energy-efficient CO2hydrogenation with fast response using photoexcitation of CO2adsorbed on metal catalysts Many heterogeneous catalytic reactions occur at high temperatures, which may cause large energy costs, poor safety, and thermal degradation of catalysts. Here, we propose a light-assisted surface reaction, which catalyze the surface reaction using both light and heat as an energy source. Conventional metal catalysts such as ruthenium, rhodium, platinum, nickel, and copper were tested for CO 2 hydrogenation, and ruthenium showed the most distinct change upon light irradiation. CO 2 was strongly adsorbed onto ruthenium surface, forming hybrid orbitals. The band gap energy was reduced significantly upon hybridization, enhancing CO 2 dissociation. The light-assisted CO 2 hydrogenation used only 37% of the total energy with which the CO 2 hydrogenation occurred using only thermal energy. The CO 2 conversion could be turned on and off completely with a response time of only 3 min, whereas conventional thermal reaction required hours. These unique features can be potentially used for on-demand fuel production with minimal energy input. Metal nanoparticles loaded onto supports have been typically used as heterogeneous catalysts for surface reactions such as hydrogenation, oxidation, reforming, and coupling reactions [1] , [2] , [3] , [4] , [5] . Surface reactions often require high temperatures to overcome the activation energy barrier. Operating the reactor at a high temperature may demand excessive energy and stringent safety controls. Recently, light-assisted surface reactions have been reported [6] , [7] , [8] , [9] , [10] , [11] . Using heat and light together as two different energy sources might minimize the overall energy usage and provide unique features, which cannot be provided by conventional thermal catalytic reactions. Enhancing the catalytic activity under light irradiation has been reported for heterogeneous reactions including ethylene epoxidation on Ag nanocubes, reverse water–gas shift reaction on Al@Cu 2 O, ethanol dehydrogenation on Ag–Ni nanosnowmans [6] , [7] , [8] . Light is absorbed on the catalyst and then transferred to reactant molecules on the surface by heat or hot electrons. The photothermal effect, in which absorbed light energy is relaxed as heat, would occur only with a very strong light that is orders of magnitude higher than the intensity of sunlight [12] , [13] , [14] , [15] . Hot electrons are generated on metal nanoparticles by an intraband or interband transition upon light absorption. Localized surface plasmon resonance (LSPR) is a typical intraband transition that can be derived from metals with high electron mobility in sp-band. Group IB metals such as Au, Ag, and Cu are representative plasmonic metals and other transition metals also can have LSPR occasionally [8] , [9] , [16] , [17] , [18] . Non-plasmonic metal nanoparticles can produce hot electrons by interband transition, in which electrons are excited from d-band to unoccupied conduction band [19] , [20] , [21] , [22] . However, light absorption by the interband transition is usually weak, and it is effective only under UV light. When the hot electrons contribute to the surface reaction, the catalytic activity for various wavelengths of incident light typically follows the trend of their light absorption spectra. With an increase in the light absorption, more hot electrons are produced, thereby enhancing the catalytic reaction further. However, this analogy might not be applicable when light is absorbed by direct excitation of the electrons located at the hybrid orbitals of a reactant adsorbed on a metal surface. When a reactant molecule is strongly adsorbed on a metal, the energy levels of electronic orbitals are rearranged. If the energy gap between the highest occupied molecular orbital (HOMO) and the lowest unoccupied molecular orbital (LUMO) is reduced, then the incident light can excite the electrons on the hybrid orbitals promoting the surface reaction [10] , [23] , [24] , [25] . Christopher et al. reported that CO oxidation in a H 2 -rich stream can be promoted by direct photoexcitation of adsorbate (CO)–metal (Pt) bonds [10] . Zhu et al. also observed selective oxidation of aliphatic alcohols on Pt or Pd nanoparticles under visible light irradiation [11] . Here, we show that CO 2 hydrogenation is enhanced on the Ru surface under light irradiation. The effects of the metal type, Ru domain size, and Ru oxidation state are evaluated. The DFT calculation is performed to investigate the changes in the energy gap between the HOMO and LUMO levels for various metals. Light irradiation reduces the reaction temperature significantly minimizing the total energy usage for CO 2 hydrogenation. Additionally, the reaction can be turned on or off in a moment, unlike the conventional thermal reaction. Enhancement in activity upon light irradiation Various metals (i.e., Ru, Rh, Pt, Ni, and Cu) were deposited on silica supports using a wet impregnation method. The TEM images of the catalysts were shown in Supplementary Fig. 1 . 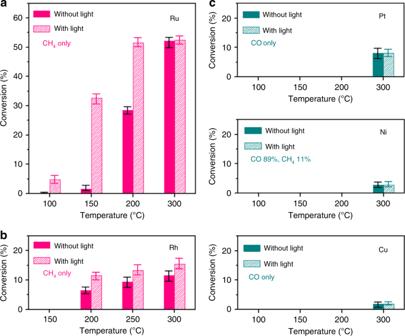Fig. 1 Light enhancement on metal catalysts. CO2conversion for CO2hydrogenation onaRu,bRh, andcPt, Ni, and Cu catalysts deposited onto silica with and without light irradiation. 0.5 vol% CO2/N2(50 sccm) and H2(1.5 sccm) was fed into the reactor through a static mixer with or without light irradiation. A Xe lamp with light intensity of 35 mW cm−2was used with a water-circulating filter to exclude any thermal effect from the light source. The error bar indicates the deviation among three independent measurements The size of the metal nanoparticles was controlled to be between 5 and 7 nm by changing the weight percentages of the metals as shown in Supplementary Table 1 . The powder catalysts containing 10 mg of metal were loaded into the custom-made photoreactor. A schematic of the reactor set-up and its photograph are shown in Supplementary Fig. 2 . 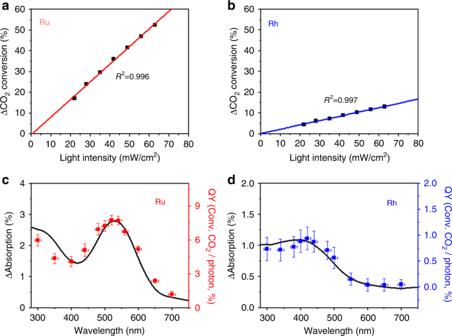Fig. 2 Dependence on light intensity and light wavelength.a,bCO2conversion for CO2hydrogenation on Ru/SiO2and Rh/SiO2when the light intensity was varied. To clarify the relation between the light intensity and CO2conversion enhanced by the light, thermal CO2conversion without light was subtracted from light-assisted CO2conversion (ΔCO2conversion). Light intensity after passing the sapphire window was measured by a spectroradiometer.c,dIn-situ UV–Vis spectroscopy in CO2flow (black lines) and quantum yield for wavelength-dependent measurement of CO2hydrogenation on Ru/SiO2or Rh/SiO2(red or blue dots). Error bars inx-direction indicates full-width at half maximum intensity of monochromatic light. Error bars iny-direction indicates a deviation among three different measurements. The in-situ UV–Vis spectroscopy and CO2conversion was measured at 150 °C for Ru/SiO2and 200 °C for Rh/SiO2 CO 2 hydrogenation was performed by flowing CO 2 and H 2 together after reducing the catalysts at 300 °C for 3 h. Figure 1 shows the CO 2 conversion data of various metals with and without light irradiation (Supplementary Table 2 for the full data). Ru and Rh produced CH 4 only, whereas Pt and Cu produced CO only. Ni produced 89% CO and 11% CH 4 . The CO 2 conversion increased upon light irradiation for Ru and Rh, while the conversion did not change for Pt, Ni, and Cu. Especially, the Ru catalyst showed remarkable enhancements. At 150 °C, the CO 2 conversion was 1.6% without light, but it increased to 32.6% with light. This conversion was obtained at 230 °C without light. By simply shining light, the reaction temperature for CO 2 hydrogenation was lowered significantly. When a higher concentration of CO 2 was used with CO 2 /N 2 /H 2 flow rates of 5/30/15 sccm, the CO 2 conversion was also significantly enhanced from 1.1 to 10.9% at 150 °C upon light irradiation as shown in Supplementary Fig. 3 . 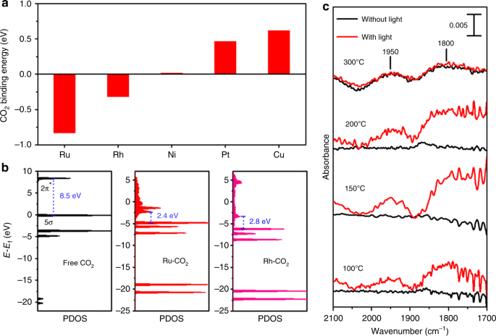Fig. 3 Binding of CO2on metal surfaces.aCO2binding energy andbHOMO-LUMO gap of free CO2, adsorbed CO2on the Ru surface, or adsorbed CO2on the Rh surface, obtained using DFT calculations.cDRIFT spectra for CO2adsorption on Ru/SiO2with or without light irradiation. 50 sccm of 0.5% CO2/N2was flowed for 10 min; the cell was purged with 60 sccm of N2for 15 min to desorb the weakly adsorbed CO2, and the IR spectra were obtained Supplementary Table 3 shows the comparison of the production rate with the literature values reported for gas-phase CO 2 hydrogenation performed under light irradiation [13] , [26] , [27] , [28] , [29] . Fig. 1 Light enhancement on metal catalysts. CO 2 conversion for CO 2 hydrogenation on a Ru, b Rh, and c Pt, Ni, and Cu catalysts deposited onto silica with and without light irradiation. 0.5 vol% CO 2 /N 2 (50 sccm) and H 2 (1.5 sccm) was fed into the reactor through a static mixer with or without light irradiation. A Xe lamp with light intensity of 35 mW cm −2 was used with a water-circulating filter to exclude any thermal effect from the light source. The error bar indicates the deviation among three independent measurements Full size image The light intensity during the CO 2 hydrogenation was 35 mW cm −2 , which is too weak to induce any photothermal effect. The photothermal effect has been observed in a light intensity range of 1–10 6 W cm −2 , regardless of the metal type [12] , [13] , [14] , [15] , [30] . The intensity of sunlight is ~100 mW cm -2 . A linear relation between the photocatalytic activity and light intensity has been well known as a fingerprint for hot electron-driven chemical reactions [7] , [8] , [31] , [32] . Figure 2a and b shows that the CO 2 conversion increased linearly as the light intensity increased on the Ru or Rh catalysts. Clearly, the light-enhanced CO 2 hydrogenation results from the hot electrons. Fig. 2 Dependence on light intensity and light wavelength. a , b CO 2 conversion for CO 2 hydrogenation on Ru/SiO 2 and Rh/SiO 2 when the light intensity was varied. To clarify the relation between the light intensity and CO 2 conversion enhanced by the light, thermal CO 2 conversion without light was subtracted from light-assisted CO 2 conversion (ΔCO 2 conversion). Light intensity after passing the sapphire window was measured by a spectroradiometer. c , d In-situ UV–Vis spectroscopy in CO 2 flow (black lines) and quantum yield for wavelength-dependent measurement of CO 2 hydrogenation on Ru/SiO 2 or Rh/SiO 2 (red or blue dots). Error bars in x -direction indicates full-width at half maximum intensity of monochromatic light. Error bars in y -direction indicates a deviation among three different measurements. The in-situ UV–Vis spectroscopy and CO 2 conversion was measured at 150 °C for Ru/SiO 2 and 200 °C for Rh/SiO 2 Full size image The silica support is photochemically inert; thus, Ru or Rh should provide hot electrons. The extent of the surface oxide was changed to observe the effect of the surface oxide for the light enhancement. While the as-made Ru/SiO 2 catalyst with a Ru size of 5.6 nm has 89% of metallic Ru and 11% of Ru oxide at the surface, the percentages of Ru oxide increased to 44 and 61% after annealing the catalyst at 500 °C in air for 1 and 60 min, respectively (Supplementary Fig. 4 ). Supplementary Fig. 5 shows the CO 2 conversion data for these samples having different amounts of Ru oxide with and without light irradiation. The enhancement from the light decreased drastically as the amount of Ru oxide increased, and the sample annealed for 60 min showed little enhancement upon light irradiation. This indicates that metallic Ru is responsible for the enhancement by light. The effect of the Ru nanoparticle size was estimated. Different sizes (2.6, 5.6, and 17.1 nm) of Ru nanoparticles were obtained by changing the weight percentages of Ru on the Ru/SiO 2 catalyst, and their TEM images are shown in Supplementary Fig. 6 . 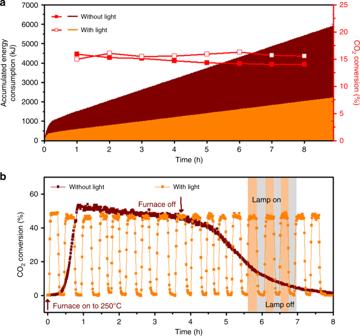Fig. 4 Energy usage and response for CO2hydrogenation with or without light irradiation.aEnergy consumption during CO2hydrogenation with or without light irradiation. The condition in which both cases showed similar CO2conversions was chosen; CO2hydrogenation occurred at 180 °C without light, or 150 °C with light. 100 mW laser (532 nm) equipped with a beam expander was used as a light source. The overall power consumption was measured by a power meter.bResponse test results for CO2hydrogenation with or without light. Att= 0, the temperature of the reactor was set at 100 °C. In the case without light, the heater was turned on, the temperature was maintained for 3 h after it reached 250 °C, and the heater was turned off. In the case with light, a Xe lamp with a light intensity of 63 mW cm−2was turned on for 15 min and turned off for 15 min repeatedly The nanoparticle sizes were checked using both powder XRD and the H 2 uptakes as shown in Supplementary Table 4 . The fraction of metallic Ru on the surface was the same as ~90%. Supplementary Fig. 7 shows that the enhancement by light was much smaller in the 2.6 nm Ru nanoparticles, while both the 5.6 and 17.1 nm Ru nanoparticles had a distinct enhancement. It was reported that larger Ru nanoparticles (e.g., ≥5 nm) exhibit a higher CO 2 conversion than smaller ones for conventional CO 2 hydrogenation because CO 2 dissociation requires higher activation barrier on smaller Ru nanoparticles [33] , [34] , [35] . Thus, we hypothesized that the enhancement by light may be related to the interaction between the Ru surface and the CO 2 molecule. Hot electrons can be produced on a metal surface by an intraband or interband transition [8] , [9] , [16] , [17] , [18] , [19] , [20] , [21] , [22] . Among Ru, Rh, Pt, Ni, and Cu, only Cu can have an intraband transition; however, the Cu catalyst did not show any enhancement for CO 2 hydrogenation under light. If hot electrons produced by the interband transition promote CO 2 hydrogenation, all the metals, not just Ru or Rh, should show an enhancement. Additionally, the interband transition is usually observed in the ultraviolet (UV) range, and the enhancement by the interband transition decreases abruptly as the wavelength of the incident light increases [20] , [22] . In-situ UV–Vis spectroscopy was performed in CO 2 flow as shown in Fig. 2c, d (black lines). While UV-DRS data (Supplementary Fig. 8 ) obtained without CO 2 showed no peak, the peaks were observed at 528 nm for Ru/SiO 2 and 410 nm for Rh/SiO 2 . When the content of Ru/SiO 2 catalyst in KBr mixture increased, the absorbance also increased without the change in peak position as shown in Supplementary Fig. 9 . Interestingly, these spectra from in-situ UV–Vis measurements (black lines) agree well with the photoaction spectra, which are the plots of quantum yield (QY) vs. wavelength (red or blue dots in Fig. 2c, d ). The QY was estimated from the CO 2 hydrogenation reaction data at each wavelength using a monochromator. Briefly, QY was calculated by dividing the number of converted CO 2 molecules with the number of incident photons at each wavelength (Supplementary Fig. 10 ). The detailed procedure is explained in Methods. The photoaction spectra also presented peaks at 520 nm for Ru/SiO 2 and 420 nm for Rh/SiO 2 . This result indicates that the hot electrons originate from light absorption by CO 2 adsorbed on the metallic Ru or Rh surface and they promote the CO 2 hydrogenation. Mechanism study The CO 2 binding energy on various metal surfaces was estimated using density functional theory (DFT) calculations, as shown in Fig. 3a . (111) surface was used for the face-centered cubic metals of Rh, Pt, Ni, and Cu, while (0001) surface was used for the hexagonal close packed metal of Ru. Various CO 2 positions were tested to obtain the minimum energy configuration as shown in Supplementary Fig. 11 . Figure 3a shows the values of the lowest CO 2 binding energy. Supplementary Fig. 12 shows the state of CO 2 with the lowest energy configurations. Ru and Rh have a negative binding energy, while Pt, Ni, Cu have a positive binding energy, indicating that CO 2 binds onto the Ru or Rh surface strongly while it does not bind to the other metal surfaces. This trend in CO 2 binding energy on various metal catalyst agrees well with CO 2 chemisorption results shown in Supplementary Table 5 and other previous report [36] . The strong adsorption of CO 2 onto the Ru or Rh surface may change the electronic structure of the CO 2 . The electronic structure of free CO 2 and CO 2 adsorbed on the metal surface were calculated, and their HOMO (5 σ bonding)–LUMO (2 π anti-bonding) gaps are shown in Fig. 3b and Supplementary Fig. 11c . The gap decreased significantly from 8.5 eV for free CO 2 to 2.4 eV for CO 2 adsorbed on the Ru surface. The energy gap of the CO 2 adsorbed on the Rh surface was 2.8 eV. These gaps are small enough for the electrons to jump under visible light irradiation. The gap was much larger as 4.5 eV for Ni, 3.8 eV for Pt, and 3.5 eV for Cu. In Fig. 2c and d , Ru had the absorption peak in the presence of CO 2 at 528 nm (~2.3 eV) and Rh had the peak at 410 nm (~3.0 eV). The calculated energy gaps of 2.4 eV for Ru and 2.8 eV for Rh are in good agreement with the experimentally obtained values. Fig. 3 Binding of CO 2 on metal surfaces. a CO 2 binding energy and b HOMO-LUMO gap of free CO 2 , adsorbed CO 2 on the Ru surface, or adsorbed CO 2 on the Rh surface, obtained using DFT calculations. c DRIFT spectra for CO 2 adsorption on Ru/SiO 2 with or without light irradiation. 50 sccm of 0.5% CO 2 /N 2 was flowed for 10 min; the cell was purged with 60 sccm of N 2 for 15 min to desorb the weakly adsorbed CO 2 , and the IR spectra were obtained Full size image The diffuse reflectance infrared Fourier transform (DRIFT) spectra for CO 2 adsorbed on the Ru surface are shown in Fig. 3c . The spectra obtained with and without light were compared. Whereas no peak appeared up to 200 °C without light, two distinct peaks were observed at 1950 and 1800 cm −1 even at 100 °C with light. The peak at 1950 cm −1 resulted from CO linearly adsorbed on Ru, and the peak at 1800 cm −1 indicated that CO was adsorbed on Ru through a bridge mode [37] , [38] . Upon light irradiation, CO 2 would be cleaved to CO ad and O ad on the Ru surface. Supplementary Fig. 13 shows the DRIFT spectra obtained when H 2 was additionally flowed after the CO 2 was adsorbed on the Ru surface. The two peaks appeared at 150 °C without light, indicating that H 2 assists in CO 2 dissociation. However, the peaks were much larger with light, confirming that light irradiation clearly promoted CO 2 dissociation. The effect of light on CO hydrogenation was also investigated. Supplementary Fig. 14a shows the CO conversion data with and without light. The CO conversion was slightly higher under light irradiation, but the differences in the conversion with and without light were rather small. Supplementary Fig. 14b shows the DRIFT spectra when CO was adsorbed on the Ru surface, and Supplementary Fig. 14c shows the DRIFT spectra when H 2 was additionally flowed after adsorbing CO onto the Ru surface. The spectra were almost identical, regardless of the light irradiation. CO hydrogenation was hardly affected by light irradiation, indicating that the enhanced activity upon light irradiation for CO 2 hydrogenation is related to the CO 2 dissociation. When CO 2 is strongly adsorbed on the Ru surface, hybrid orbitals are formed with a much shorter energy gap. If the light can easily excite the electrons in the bonding orbitals to anti-bonding orbitals, then CO 2 can be dissociated to CO. Further hydrogenation would produce CH 4 . Kinetic analysis of light-assisted CO 2 hydrogenation was performed with various CO 2 partial pressures and temperatures. Supplementary Fig. 15a shows the dependences of CO 2 conversion rates on the partial pressure of CO 2 . The CO 2 conversion rate increased as the CO 2 partial pressure increased, and reached a plateau at 4 kPa of CO 2 . The CO 2 conversion rate followed the identical saturation behaviors under light irradiation, reaching the plateau at the same CO 2 partial pressure. It indicates that the light irradiation did not change CO 2 coverage on Ru surface, but interfere with the adsorbed CO 2 species. The temperature dependence of CO 2 hydrogenation around 150 °C was investigated as shown in Supplementary Fig. 15b . Without light, the effective energy barrier ( E a ) of Ru catalyst was 70.4 kJ mol −1 , which agrees well with previous studies [39] , [40] . However, the E a decreased significantly to 36.2 kJ mol −1 with light irradiation. The incident light lowers the effective energy barrier on Ru catalyst for CO 2 hydrogenation. Comparing energy usage for thermal vs. light-assisted reactions The same CO 2 conversion can be achieved at a lower temperature with light. If the power required to shine light is less than the power required to heat the reactor, the overall energy consumption would be reduced. Figure 4a shows the total energy consumption for CO 2 hydrogenation with and without light. The reactor temperature was set to be 180 °C for the case without light, and 150 °C for the case with light. The CO 2 conversion was maintained at ~15% for both cases. The total electric power consumed was measured by an online power meter. To minimize the energy consumption for shining a light, a compact laser with a wavelength of 532 nm was used with a beam expander instead of a Xe lamp. For a CO 2 hydrogenation reaction for 8 h, the total energy consumption was 5411 kJ for the case without light, and 2020 kJ for the case with light. Only 37% of the energy was consumed when light was irradiated together. Clearly, the energy required for catalytic reactions in a continuous flow reactor can be significantly reduced by light irradiation. Fig. 4 Energy usage and response for CO 2 hydrogenation with or without light irradiation. a Energy consumption during CO 2 hydrogenation with or without light irradiation. The condition in which both cases showed similar CO 2 conversions was chosen; CO 2 hydrogenation occurred at 180 °C without light, or 150 °C with light. 100 mW laser (532 nm) equipped with a beam expander was used as a light source. The overall power consumption was measured by a power meter. b Response test results for CO 2 hydrogenation with or without light. At t = 0, the temperature of the reactor was set at 100 °C. In the case without light, the heater was turned on, the temperature was maintained for 3 h after it reached 250 °C, and the heater was turned off. In the case with light, a Xe lamp with a light intensity of 63 mW cm −2 was turned on for 15 min and turned off for 15 min repeatedly Full size image In a thermally heated reactor, controlling the temperature instantaneously is nearly impossible. Figure 4b shows the response in CO 2 conversion for turning on or off the heater or light source. When the heater was turned on at t = 0, it took 52 min to reach the target temperature of 250 °C and the highest conversion. More importantly, cooling down the reactor took much longer time. After the heater was turned off at t = 3.8 h, CO 2 conversion was still observed with a long tail due to the residual heat in the reactor. However, the response became much faster with light irradiation. The highest conversion was immediately obtained after turning on the lamp. The CO 2 conversion dropped to 0% within 3 min after turning off the lamp. The instantaneous control of CO 2 conversion cannot be achieved with a conventional thermal reactor. This unique feature might be useful for on-demand CH 4 production. CO 2 hydrogenation was performed on metallic catalysts of Ru, Rh, Pt, Ni, and Cu with and without light irradiation. The CO 2 conversion was enhanced significantly on a Ru catalyst by light irradiation. The CO 2 conversion was 1.6% at 150 °C without light on Ru, but the conversion increased to 32.6% at 150 °C with light. The effects of the Ru surface oxidation state and Ru nanoparticle size were evaluated. The light-enhancement appeared only at the metallic Ru surface, and larger nanoparticles exhibited more enhancement. Hot electrons generated upon light irradiation enhanced the CO 2 conversion; however, the enhancement was not related to the light absorption on the metal surface. Rather, it was related to the HOMO-LUMO energy gap of the CO 2 adsorbed on the metal surface. DFT calculations showed that CO 2 is strongly bound to the Ru surface, and the energy gap is reduced from 8.5 eV in free CO 2 to 2.4 eV in CO 2 adsorbed on the Ru surface. Especially, light promotes CO 2 dissociation to CO as confirmed by the DRIFTS data. Light irradiation could lower the reaction temperature for CO 2 hydrogenation. When total energy consumption was compared at a CO 2 conversion rate of 15%, the energy required for the case with light irradiation was only 37% of that for the case without light irradiation. Furthermore, the CO 2 conversion could be instantaneously turned on and off by light irradiation unlike a conventional thermal reaction. This light-assisted heterogeneous reaction can contribute to lowering energy consumption in chemical production, with a much faster response for the changes in the reaction condition. Catalyst synthesis Metal nanoparticle catalysts supported on silica (M/SiO 2 , M = Pt, Ni, Cu, Ru, and Rh) were prepared using a wet impregnation method. Different amounts of metal precursors, (metal acetylacetonates; details in Supplementary Table 1 ) were dissolved in acetone (10 mL, Sigma-Aldrich) and added to silica nanopowder (1 g, Sigma-Aldrich). The slurry mixture was dried at 80 °C for 30 min, and it was placed into the furnace and heated up to 300 °C with a ramping rate of 10 °C min -1 in 10 vol% H 2 /N 2 (200 sccm). Then, catalysts were reduced at 300 °C for 3 h. The extent of the surface oxidation on Ru/SiO 2 was controlled by oxidizing the catalyst at 500 °C under static air for various treatment times (1 or 60 min). CO 2 hydrogenation The M/SiO 2 (M = Pt, Ni, Cu, Ru, and Rh) catalysts were placed in a cylindrical quartz sample holder (2 cm of diameter). Metal 10 mg was loaded for all the reactions. The sample holder was placed in a customized photoreactor equipped with a sapphire glass window (a thickness of 23 mm) as shown in Supplementary Fig. 2 . It should be noted that a water circulating filter was located in front of the Xe lamp (300 W, Newport) to exclude the effect of thermal radiation from the lamp. The catalysts were reduced prior to the CO 2 hydrogenation for 3 h at 300 °C under 10 vol% H 2 /N 2 flow. In a typical CO 2 hydrogenation, a mixture of 0.5 vol% CO 2 /N 2 (50 sccm) and H 2 (1.5 sccm) was fed into the reactor through a static mixer with or without light irradiation at atmospheric pressure. The CO 2 conversion was monitored by an online gas chromatograph (YL6100 GC, YL Instrument) equipped with molesieve/PORAPAK N columns (Sigma-Aldrich), a thermal conductivity detector (for H 2 and N 2 detection), and a flame ionization detector (for CH 4 , CO, and CO 2 detection) with a methanizer. Quantitative analysis was performed using N 2 as an internal standard. The dependency on the light intensity or light wavelength was measured at 150 °C for Ru and 200 °C for Rh. The light intensity was varied by changing the electric power of the lamp and measured by a spectroradiometer (CS2000, KONICA MINOLTA). The transmittances of the liquid filter and the sapphire glass window are shown in Supplementary Fig. 16a, b . The light intensity was corrected excluding the effect of the liquid filter and the sapphire glass window. The photoaction spectra were obtained using a monochromator (MonoRa151i, Dongwoo Optron) with wavelengths shown in Supplementary Fig. 16c . A 532 nm laser (100 mW, CNI laser) was used as the light source for the energy consumption test. Estimation of the QY The energy of the irradiated light for a given time is: 
    E = nhc/λ = IAs,
 (1) where n is a number of incident photon, λ is a wavelength of incident photon, h is Planck constant, c is a speed of light, I is the light intensity, A is the area of irradiation, and s is irradiation time. Then incident photon flux is defined as: 
    n/s = E/sλ/hc = IAλ/hc. (2) The QY can be estimated as: 
    QY = n_CO_2/s/n/s,
 (3) where \(n_{{\mathrm{CO}}_2}\) is the number of the converted CO 2 molecules. The wavelength-dependent measurement was performed using a monochromator (MonoRa151i, Dongwoo Optron). In prior to the measurement, the monochromatic light was calibrated with a spectrometer (Maya 2000 Pro, Ocean Optics) as shown in Supplementary Fig. 16c . The intensity of the monochromatic light was measured with an optical power meter (PM204, Thorlab) after the monochromatic light passed through a sapphire window of the reactor. The catalytic activity under the monochromatic light irradiation was measured at steady state for CO 2 hydrogenation. The rate of the CO 2 molecules converted by the incident photon was estimated excluding the CO 2 conversion from thermal reaction. Characterizations The morphology of prepared catalysts was observed using HR-TEM (TECNAI). A powder X-ray diffractometer (SmartLab, RIGAKU) was used to determine the crystalline size of the metal nanoparticles. X-ray photoelectron spectroscopy (XPS, Thermo VG Scientific) equipped with a monochromatic Al Kα X-ray source was used to measure the surface properties of metal nanoparticles. The binding energies were calibrated with adventitious C 1 s signal at 285 eV as a reference. The absorption spectra of the metal catalysts were obtained using an UV-diffuse reflectance spectrometer (UV-DRS) (UV3600, Shimadzu). Elemental analysis was conducted using an inductively coupled plasma optical emission spectrometer (ICP-OES 720, Agilent) to confirm the actual metal content in the M/SiO 2 catalysts. In situ diffuse reflectance infrared Fourier transform spectroscopy (DRIFTS) measurements were performed using a FT-IR spectrometer (Thermo, Nicolet 6700) equipped with a MCT detector. In situ UV–Vis spectroscopy was performed using a UV–Vis spectrophotometer (Perkin Elmer, lambda 1050) equipped with diffuse reflectance accessory (PIKE, DiffuseIR) enabling gas flow and temperature control. The power consumption during the CO 2 hydrogenation was monitored using a 2-channel power meter (WT500, YOKOGAWA) which contacted both furnace and light sources. The energy consumption by the standby power was excluded for both cases. Theoretical calculation using DFT All of the quantum chemical calculations were performed with the Vienna ab initio simulation package [41] . We used the projector augmented wave pseudopotentials with Perdew–Burke Ernzerhof [42] exchange correlation functional. The energy cutoff was set as 500 eV, while a 5 × 5 × 1 k -point grid was used for energy relaxation, and 20 × 20 × 1 for the density of states calculation using the Monkhorst–Pack scheme [43] . Five metal catalysts (Cu, Ni, Pt, Rh, and Ru) were modeled using four layered slabs with the surfaces of (111) used for Cu, Ni, Pt, and Rh, and (0001) for Ru with a 15 Å vacuum region. Only the atoms from the top layer could relax during the DFT simulations. The CO 2 molecules were initialized on different atomic sites (Supplementary Fig. 11 ), and the binding energy was determined by the lowest energy configurations (Supplementary Fig. 12 ). The angles of the CO 2 molecules are slightly bent due to the strong interaction between the metal surfaces and the CO 2 molecule. The CO 2 binding energy was defined as follows: 
    E_bind = E_catalyst + CO_2 - (E_catalyst + E_CO_2),
 (4) where \(E_{{\mathrm{bind}}}\) is the binding energy of CO 2 on the metal catalyst, and \(E_{{\mathrm{catalyst}} + {\mathrm{CO}}_2}\) is the total energy of the metal catalyst with a single CO 2 molecule. \(E_{{\mathrm{catalyst}}}\) and \(E_{{\mathrm{CO}}_2}\) are the total energy of free metal catalyst and CO 2 molecule, respectively. Data availability The authors declare that the data supporting the findings of this study are available within the paper and its Supplementary Information files.